A general and scalable synthesis approach to porous graphene Porous graphene, which features nano-scaled pores on the sheets, is mostly investigated by computational studies. The pores on the graphene sheets may contribute to the improved mass transfer and may show potential applications in many fields. To date, the preparation of porous graphene includes chemical bottom-up approach via the aryl–aryl coupling reaction and physical preparation by high-energy techniques, and is generally conducted on substrates with limited yields. Here we show a general and scalable synthesis method for porous graphene that is developed through the carbothermal reaction between graphene and metal oxide nanoparticles produced from oxometalates or polyoxometalates. The pore formation process is observed in situ with the assistance of an electron beam. Pore engineering on graphene is conducted by controlling the pore size and/or the nitrogen doping on the porous graphene sheets by varying the amount of the oxometalates or polyoxometalates, or using ammonium-containing oxometalates or polyoxometalates. Various kinds of methods have been developed to prepare graphene sheets, such as chemical vapour deposition [1] , [2] , epitaxial growth of graphene films [3] , bottom-up synthesis [4] , [5] and reduction of graphene oxide (GO) [6] , [7] . In these methods, reduction of GO is a frequently used method for material scientists to obtain graphene [8] , [9] , and graphene-based materials and devices [10] , [11] , [12] . Chemical oxidation and exfoliation of graphite produce GO at gram scale, and introduce a large amount of oxygen-containing groups and defects in the graphene sheets [7] , [13] . Reduction through chemical, thermal and electrochemical approaches could remove most of the oxygen-containing groups, but the defects usually retain in the reduced GO (RGO) sheets [5] , [6] , [14] . Since the report on peeled-off graphene in 2004 (ref. 15 ), many researchers attempted to find approaches to repair the defects in the RGO and make the performance infinitely close to the perfect pristine graphene, especially its electronic properties [16] , [17] . However, subsequent research has been focused on the potential applications arising from the defects in the graphene sheets from a material science perspective. Huang and co-workers [18] recognized the defective nature of GO, and increased the amount of defects in the GO through steaming etching method. The steam-etched porous GO showed great improvement in the NO 2 sensing. Despite of the sp 3 -carbon domains on the RGO sheet, defects in the RGO are pores of different sizes and shapes, therefore, it could be considered as a kind of porous graphene (pGRF). pGRF, which is a derivative of graphene with nano-scaled pores on the sheets, was mostly studied in the computational and physical fields [19] . Owing to the pores on the graphene sheets, the rate of mass transfer is improved; therefore, pGRF exhibits distinct properties from pristine graphene that leads to its potential applications in numerous fields, such as gas separation and purification [20] , water desalination [21] , ion channel [22] and DNA sequencing [23] . pGRF has been prepared by helium ion bombardment [24] , electron beam irradiation [25] and laser irradiation [26] , in which the high-energy media, such as electron and laser, are used to produce pores on single graphene sheet, and the pore size ranges from atomic precision (<1 nm) to nano-scaled dimension (~1–500 nm). Chemical methods have also been developed to prepare pGRF in recent years, such as bottom-up synthesis and stream etching. Regular two-dimensional (2D) polyphenylene network, which possesses periodic conjugated structure with missed phenyl ring and could be considered as order-structured pGRF, was synthesized through aryl−aryl coupling reaction of well-designed molecular building blocks (macrocycle cyclohexam-phenylene) on the Ag surface [27] , [28] . As the previous methods mentioned above, pGRF are prepared on substrates and the yield is counted in terms of number of ‘pieces’; furthermore, high-cost electron-based instruments are usually needed. Therefore, the studies of pGRF are usually carried out as a kind of nanodevice and in computational chemistry owing to the lack of an effective synthesis method with bulk production [19] . As for the commercial application of a newly developed material, the production at large scale with low cost is the last bottleneck. Therefore, it is essential to explore economical methods for the synthesis of pGRF for the experimental investigation on its chemical and physical properties [9] . Carbothermal reactions are thermal reactions that use carbon as the reducing agent at high temperature [29] , [30] , [31] , in which most metal oxide could be reduced into metal and metal carbide accompanying with the carbon atom leaving in the form of carbon monoxide and carbon dioxide [32] . The most prominent example is that of iron ore smelting, which is used in the production of iron or steel. Graphene, GO and RGO are 2D carbon nanomaterials with which the carbothermal reaction would happen at a relatively low temperature owing to their high surface energy. Herein, we demonstrate a general and scalable synthesis approach to pGRF through carbothermal reaction by using GO as graphene sources etched by oxometalates (OM) or polyoxometalates (POM). Owing to the carbothermal reaction between carbon atoms of graphene and the metal oxide nanoparticles generated from OM or POM, nano-scaled (1–50 nm) pores are generated on the graphene sheets. After the removal of the metal oxides containing species by treatment with acid, pGRF could be obtained. In addition, the formation process of pores is observed in situ with the assistance of electron beam in the high-vacuum scanning electron microscope chamber. Meanwhile, pore engineering on graphene is conducted by controlling the pore size and the nitrogen doping on the pGRF sheets. The pore size on the pGRF sheets could be controlled by the amount of the OM or POM in the precursor, and nitrogen-doped pGRF could be prepared by using ammonium-containing OM or POM. Pore formation on graphene Pore formation on graphene was conducted through a carbothermal reaction by using the metal oxide nanoparticles obtained in situ as the nano-scale etcher ( Fig. 1 ). In the thermal reaction, OM or POM could be thermally decomposed into metal oxide nanoparticles [33] , [34] that adsorbed on the surface of RGO sheets [35] and oxidized the neighbour carbon atoms on RGO into carbon dioxide or carbon monoxide [36] , therefore, pores or defects generated on RGO sheet. As shown in the scanning electron microscopy (SEM) image of GOM (the composite of RGO and the thermal-generated metal oxide nanoparticles; Fig. 1 and Supplementary Fig. 1b ), nano-scaled pores could be observed under nanoparticles, validating the pore generation through the etching by the metal oxide nanoparticles. pGRF could be obtained after the removal of the metal-containing species by immersing the GOM samples in the aqueous acid solution (HCl, 1.0 M ) for a week. 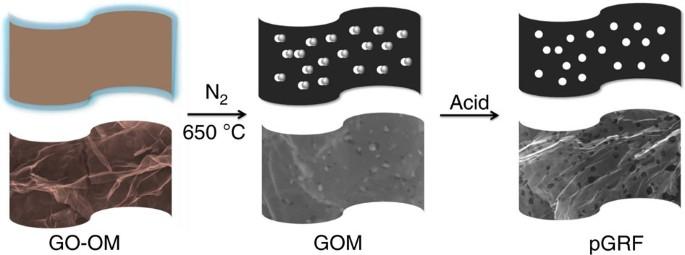Figure 1: Illustration of the synthesis process of pGRF. During the thermal reaction, the adsorbed OM or POM thermally decomposes into metal oxide nanoparticles, which are the nano-scale etcher of the TRG to produce pGRF in the carbothermal process. Figure 1: Illustration of the synthesis process of pGRF. During the thermal reaction, the adsorbed OM or POM thermally decomposes into metal oxide nanoparticles, which are the nano-scale etcher of the TRG to produce pGRF in the carbothermal process. Full size image Various kinds of OM and POM could be used to prepare pGRF samples, and the pores formed on the pGRF sheets could be observed directly by SEM and transmission electron microscopy (TEM). 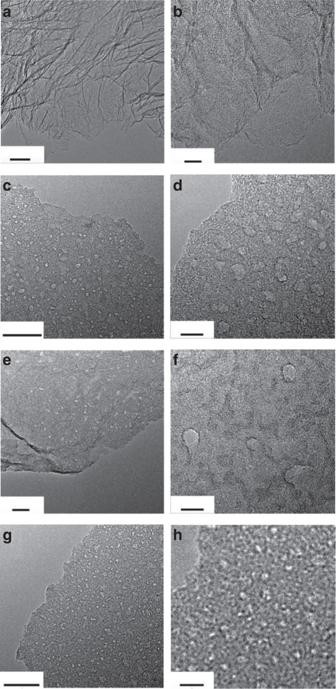Figure 2: TEM images of TRG and the pGRFs prepared using different OMs or POMs. TRG (a,b), pGRF-W (c,d), pGRF-Mo (e,f) and pGRF-Ti (g,h). Scale bars, 50 nm (a,c,e,g) and 10 nm (b,d,f,h). Figure 2 and Supplementary Fig. 2 shows the TEM images of pGRF samples prepared by using different OM (Na 2 MoO 4 , Na 2 WO 4 , NaAlO 2 , Na 2 SnO 3 , K 2 TiO 3 , KMnO 4 or Na 3 VO 4 ) or POM ((NH 4 ) 6 Mo 7 O 24 or H 3 PMo 12 O 40 ) as etcher, and the as-prepared pGRF samples show nano-scaled pores of ~1–10 nm on the sheet. The pore sizes on pGRF-W, pGRF-Mo, pGRF-Mn, pGRF-Sn, pGRF-Ti, pGRF-Mo/N and pGRF-Mo/P are ~1–10 nm, and are ~1–5 nm on pGRF-Al and pGRF-V. Figure 2: TEM images of TRG and the pGRFs prepared using different OMs or POMs. TRG ( a , b ), pGRF-W ( c , d ), pGRF-Mo ( e , f ) and pGRF-Ti ( g , h ). Scale bars, 50 nm ( a , c , e , g ) and 10 nm ( b , d , f , h ). Full size image Another evidence for the introduction of pores on graphene sheets is the change of the D / G intensity ratio ( Supplementary Fig. 3 ). In the Raman spectra of carbon materials, D - ( ca . 1,350 cm −1 ) and G - (ca. 1,590 cm −1 ) bands are characteristic signals [37] . In the graphene-based materials, G -band is corresponding to the sp 2 -hybridized carbon atoms in the hexagonal framework, and D -band is indicative of sp 3 -hybridized carbon atoms on the defects and edges of the graphene sheets [7] , [38] . The pGRF samples exhibit larger D / G intensity ratio compared with the values of GO and thermal RGO (TRG). In the carbothermal etching of graphene, more defects and edges are introduced on graphene sheets, resulting in the increase in the amount of the sp 3 -hybridized carbon atoms, therefore, the D -band intensity increased in the pGRF samples. Fourier transform infrared (IR) spectra ( Supplementary Fig. 4 ) confirms that the disappearance of carbonyl signal from GO to TRG, and also appearance of a tiny carbonyl signal in pGRF samples. Furthermore, the etching on graphene sheets also caused an increase in the oxygen content of pGRF-Mo (11.56 at %, at % means atomic percentage) compared with that of TRG (6.98 at %) ( Supplementary Fig. 5 and Supplementary Table 1 ). The transformation of the OM or POM was studied by X-ray diffraction (XRD) analysis. In the carbothermal reaction, the carbon atoms on the TRG sheets were partially oxidized into carbon dioxide and/or carbon monoxide and left the graphene sheet, and the OM or POM species was decomposed and reduced into metal oxide, metal and/or even metal carbide compounds ( Supplementary Figs 6 and 7 and reaction equations (1) and (2)). For OM or POM salts containing sodium or potassium, the final product also includes sodium carbonate or potassium carbonate. The signals of Na 2 MoO 4 , MoO 2 , MoO 3 and Na 2 CO 3 could be observed in the XRD pattern of GOMo ( Supplementary Fig. 7a ), whereas, the signals of K 2 Ti 6 O 13 , TiO 2 , Ti 3 O 5 , TiC and K 2 CO 3 could be observed in the XRD pattern of GOTi ( Supplementary Fig. 7b ). For OM or POM containing ammonium, the product also included ammonia. In the preparation of pGRF using ammonium molybdate as etcher, ammonium molybdate was thermally decomposed into molybdenum oxide and ammonia. In the carbothermal reaction, the molybdenum oxide containing nanoparticles were reduced by the carbon atoms on graphene sheets ( Supplementary Figs 7c and 8 ), and the molybdenum oxide species is mainly in the form of MoO 2 in the sample. In situ observation of the pore formation In order to validate the pore generation process, etching of the graphene film was conducted in the SEM chamber for observation of the pore formation process in situ , in which the high-voltage electron was used as the energy and electron provider ( Fig. 3 ). GO film on silicon wafer was prepared by drop-coating method and then thermally reduced into TRG film. Aqueous ammonium molybdate solution (0.1 ml) was then dropped on the TRG film and was gradually assembled into particles on the TRG film after kept quiescent at 40 °C. The assembly of ammonium molybdate is investigated by SEM at a voltage of 1.0 KV, and it is found that the concentration of the aqueous ammonium molybdate solution is very important for the controlling of the particle size assembling on the TRG film. The particle size increases when the concentration of the ammonium molybdate solution increases from 0.1, 1.0 to 10 m M . When the concentration is 0.1 m M , the ammonium molybdate nanoparticles assemble uniformly on the TRG film and the particle size is ~10–20 nm. When the concentration increased to 1.0 and 10.0 m M , the particles become larger, which are 50–100 and 200–300 nm, respectively ( Fig. 3 ). 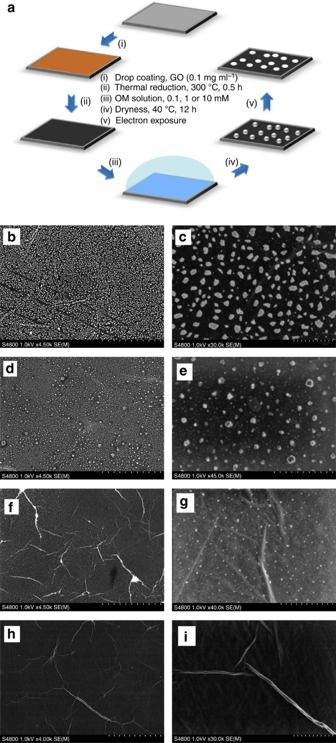Figure 3: The carbothermal etching process on graphene film and SEM images. (a) Schematic illustration of carbothermal etching process. (b–i) SEM images of the assembly of OM on the TRG film prepared at different concentrations of the aqueous ammonium molybdate solution: 10.0 mM (b,c), 1.0 mM (d,e), 0.1 mM (f,g) and 0 mM (h,i). Scale bars, 10.0 μm (b,d,f,h) and 1.0 μm (c,e,g,i). Figure 3: The carbothermal etching process on graphene film and SEM images. ( a ) Schematic illustration of carbothermal etching process. ( b – i ) SEM images of the assembly of OM on the TRG film prepared at different concentrations of the aqueous ammonium molybdate solution: 10.0 mM ( b , c ), 1.0 mM ( d , e ), 0.1 mM ( f , g ) and 0 mM ( h , i ). Scale bars, 10.0 μm ( b , d , f , h ) and 1.0 μm ( c , e , g , i ). Full size image The creation of pores on the TRG film was conducted in the high-vacuum chamber of SEM with the assistance of the electron beam, and the process was observed in situ as shown in Fig. 4 and the Supplementary Movie 1 . The SEM images were recorded every minute, and the wrinkles on TRG were used as the mark for the investigation. The voltage of the electron beam increases to 2.0 KV and the whole etching process needs only 3–5 min depending on the voltage. When exposed to the electron beam, the ammonium molybdate nanoparticles gradually disappear and finally pores appear on the TRG sheets after ~3 min ( Fig. 4d ). The high energy of electron beam provides enough energy for the decomposition of ammonium molybdate into molybdenum oxide and the carbothermal reaction between the molybdenum oxide and graphene sheets. Molybdenum oxide is a good redox catalyst, therefore, the electron would also promote the carbothermal reaction. Finally, the resulted MoO 3 was sublimated in the high-vacuum and high-voltage chamber. The continuous observation is shown in Supplementary Movie 1 , in which the whole process of the pore formation was recorded. 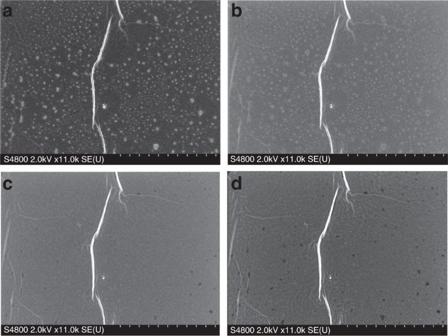Figure 4: SEM observation of the pore formation process. SEM images of TRG-OMo/N film before (a) and after electron exposure at different stages: (b) 1 min, (c) 2 min and (d) 3 min. Scale bar, 5.0 μm. Figure 4: SEM observation of the pore formation process. SEM images of TRG-OMo/N film before ( a ) and after electron exposure at different stages: ( b ) 1 min, ( c ) 2 min and ( d ) 3 min. Scale bar, 5.0 μm. Full size image Pore size control on pGRF The pore size could be controlled by the particle size of the metal oxide nanoparticles adsorbed on the GO sheets, which is absolutely tuned by the amount of OM or POM in the GO-OM precursor. (NH 4 ) 6 Mo 7 O 24 was used as the etcher for the pore size control experiments, and pGRF-Mo/N-1 and pGRF-Mo/N-2 were prepared by varying the weight ratio of the GO to ammonium molybdate, which are 1:1 and 1:2, respectively. The relative products were named as sample-1 (GO-OMo/N-1 and GOMo/N-1) and sample-2 (GO-OMo/N-2 and GOMo/N-2). As the TEM and SEM images shown in Fig. 5 and Supplementary Fig. 1 , the pore size of pGRF-Mo/N-1 is smaller than that of pGRF-Mo/N-2. The pore produced on pGRF-Mo/N-1 is ~5–10 nm ( Fig. 5a,b ), and is ~20–50 nm on the pGRF-Mo/N-2 ( Fig. 5c,d ). The ammonium molybdate species was well dispersed in the homogeneous GO-OMo/N precursor, therefore, the concentration of the ammonium molybdate in the GO-OMo/N matrix is different with varying the amount of ammonium molybdate added to a same amount/volume of GO dispersion. During the thermal reaction, the sizes of the as-formed molybdenum oxide nanoparticles are different depending on the amount of ammonium molybdate, and the pore size on the pGRF could be determined by the molybdenum oxide nanoparticles. pGRF-Mo/N-2 exhibits larger D / G intensity ratios as compared with pGRF-Mo/N-1 in the Raman spectra ( Supplementary Fig. 3b ), indicating that pGRF-Mo/N-2 contains more sp 3 -hybridized carbon atoms and/or defects than pGRF-Mo/N-1. 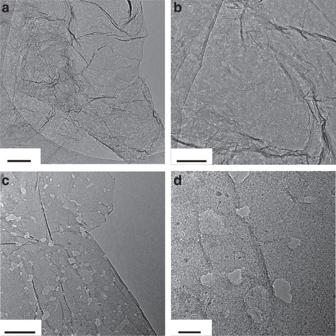Figure 5: pGRF-Mo/N-1 and pGRF-Mo/N-2 prepared with different OM amounts. TEM images of pGRF-Mo/N-1:a(scale bar, 200 nm) andb(scale bar, 100 nm); and pGRF-Mo/N-2:c(scale bar, 100 nm) andd(scale bar, 20 nm). Figure 5: pGRF-Mo/N-1 and pGRF-Mo/N-2 prepared with different OM amounts. TEM images of pGRF-Mo/N-1: a (scale bar, 200 nm) and b (scale bar, 100 nm); and pGRF-Mo/N-2: c (scale bar, 100 nm) and d (scale bar, 20 nm). Full size image Nitrogen-doped pGRF Elements in the third or fifth group are usually used as the doping atoms, such as nitrogen and boron atoms [39] , [40] . In the preparation of the pGRF using ammonium molybdate as etcher, we found the pGRF sample was nitrogen doped. Ammonia is a frequently used nitrogen-doping agent in the preparation of nitrogen-doped graphene-based materials and devices [41] , and ammonium molybdate can be thermally decomposed at different temperature to generate ammonia (equations (3, 4, 5) and Supplementary Fig. 8 ) [33] , [34] , which serves as the nitrogen precursor for the nitrogen doping of the pGRF samples. The C−N formation is validated by the X-ray photoelectron spectroscopy (XPS) spectra, and the nitrogen content in the pGRF-Mo/N-1 sample increases to 4.54 at % ( Supplementary Fig. 5 and Supplementary Table 1 ), which is comparable to the NH 3 -assisted nitrogen-doping method [40] , [41] . Further analysis of the N 1s region shows that the C−N could be divided into four kinds ( Fig. 6 ): quaternary N (~23.29 at %), pyrrolic N (~45.68 at %), pyridinic N (~23.48 at %) and amino N (~7.55 at %), and about half of the C−N is attributed to the pyrrolic N atoms [39] . Another evidence of the nitrogen doping is the IR spectra ( Supplementary Fig. 9 ), in which the absorption peak of the carbon skeleton shifts from 1,565 cm −1 in pGRF-Mo-1 to 1,575 cm −1 in pGRF-Mo/N-1 (refs 33 , 34 ). The hypsochromic/blue shift (~10 cm −1 ) might be owing to the change of the electron density for the conjugated system of the pGRF sheet after nitrogen doping [33] , [34] . Chemical doping is an important approach to enhance the electrical properties of graphene, and the nitrogen-doped pGRF would have better performance in electrochemical areas owing to the change in the electrical properties. 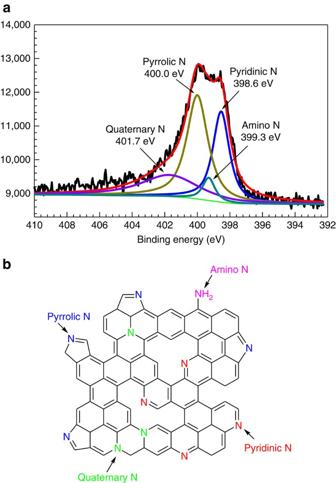Figure 6: XPS analysis of pGRF-Mo/N-1. (a) XPS spectrum of pGRF-Mo/N-1 (N1sregion). (b) Illustration of different kinds of nitrogen atoms in pGRF-Mo/N-1. Figure 6: XPS analysis of pGRF-Mo/N-1. ( a ) XPS spectrum of pGRF-Mo/N-1 (N 1s region). ( b ) Illustration of different kinds of nitrogen atoms in pGRF-Mo/N-1. Full size image There are two kinds of pore in the pGRF samples: pores on the sheets and pores/spaces between sheets. The pores on the sheets are formed via metal oxide nanoparticle etching that results in the vacancies formation via release of carbon monoxide or dioxide and/or hole formation. In the meanwhile, the interlayer pores/spaces are formed via the assembly of pGRF sheets. TRG materials always possess high surface area owing to the expansion during the thermal reduction of GO, in which the oxide functionalities were striped through the extrusion of carbon oxide and water molecules, which expanded the space between graphene sheets, therefore, high surface area would be obtained for TRG materials. In our experiment, TRG possesses a surface area of ~430 m 2 g −1 and pore volume of 1.08 cm 3 g −1 ( Supplementary Fig. 10 and Supplementary Table 2 ). The RGO sheets tend to partially restack together to form aggregates containing several layers of graphene. This is the reason that TRG show a much lower specific surface area than the theoretical value of graphene (2,600 m 2 g −1 ). pGRF samples also possess high surface area of ~400 m 2 g −1 ( Supplementary Fig. 10 and Supplementary Table 2 ), which is mainly contributed by the porosity between pGRF sheets ( Fig. 7a ). Besides the pores/spaces between the pGRF sheets, the pores on the pGRF sheets ( Fig. 7b ) enable the mass transport through the pGRF sheets in a 3D model owing to the nano-scale pores on the sheets, therefore, the mass transfer path could be shorten and the performance would be enhanced. However, mass are mainly transporting in a 2D model along the space between the graphene sheets in the TRG samples, because the direction vertical to the graphene sheets is blocked by the micrometer-scaled graphene sheets. 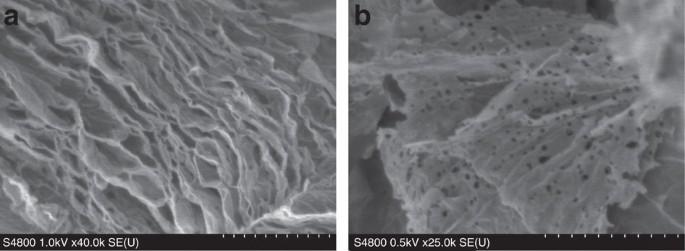Figure 7: SEM images of the pGRF samples. (a) Side view, scale bar, 1.0 μm. (b) Top view, scale bar, 2.0 μm. Figure 7: SEM images of the pGRF samples. ( a ) Side view, scale bar, 1.0 μm. ( b ) Top view, scale bar, 2.0 μm. Full size image The pore engineering on graphene sheets through carbothermal reaction provides a general and cost-effective method for the synthesis of pGRF. This scalable synthesis method should allow studies of pGRF to be advanced from computational studies and device fabrication to materials construction and applications. On the basis of the carbothermal reaction and the synthesis experience of graphene−metal oxide composites, various kinds of metal oxide nanoparticles could be used as the etchers. Owing to the pores on the pGRF sheet, pGRF shorten the mass transfer path and would have enhanced performance in the application related to mass transfer. Materials Natural flake graphite with an average particle diameter of 20 μm (99 wt% purity) was obtained from Yingshida Graphite Co. Ltd, Qingdao, China. Sulphuric acid (98 wt%), hydrogen peroxide (30 wt%), sodium nitrate and ethanol were purchased from Beijing Chemical Works, China. Sodium molybdate hydrate (Na 2 MoO 4 ·2H 2 O, OMo), sodium tungstate hydrate (Na 2 WO 4 ·2H 2 O, OW), sodium aluminate (NaAlO 2 , OAl), sodium stannate hydrate (Na 2 SnO 3 ·3H 2 O, OSn), potassium titanate (K 2 TiO 3 , OTi), sodium orthovanadate hydrate (Na 3 VO 4 ·12H 2 O, OV), ammonium molybdate hydrate ((NH 4 ) 6 Mo 7 O 24 ·4H 2 O, OMo/N), phosphomolybdic acid (H 3 PMo 12 O 40 , OMo/P), molybdenum dioxide, molybdenum trioxide and potassium permanganate (KMnO 4 , OMn) were purchased from Sinopharm Chemical Reagent Co. Ltd, China. All these reagents were of reagent grade and used without further purification. Ultrapure water (18.2 MΩ cm) was obtained by the Millipore−ELIX water purification system. Preparation of pGRF pGRF was prepared by using OM (M=Mo, W, Al, Mn, Sn, Ti or V) as the etching agents. Aqueous GO dispersion was prepared by the modified Hummers’ method [42] , [43] . OM (1.13 mmol) was added into aqueous GO dispersion (4 mg ml −1 , 50 ml), and the mixture was sonicated for 0.5 h and was stirred overnight. The homogeneous mixture was freeze-dried to obtain solid GO-OM, which was then heated at a rate of 10 °C min −1 to 650 °C for 2 h and cooled down to room temperature in the atmosphere of nitrogen. The obtained black product, named as GOM, was immersed in aqueous HCl solution (1 M ) and stirred for a week to remove the metal-containing species, such as metal oxides. Finally, pGRF sample was collected by filtration, washing with water and ethanol, and drying at 60 °C in vacuum. The final product was named as pGRF-M (M=Mo, W, Al, Mn, Sn, Ti or V). POM, such as OMo/N and OMo/P, could also be used to prepare pGRF with the same condition mentioned above, and the relative samples were named as GO-OMo/N or GO-OMo/P, GOMo/N or GOMo/P, and pGRF-Mo/N and pGRF-Mo/P. Freeze-dried GO was thermally decomposed at 650 °C for 2 h with the same condition mentioned above, and the product was named as TRG. Carbothermal etching on graphene film Aqueous GO dispersion spinning coated on silicon wafer [44] , and was then thermally reduced at 300 °C for 30 min in the atmosphere of nitrogen. Aqueous OMo/N solution (0.1, 1.0 or 10.0 mM, 0.1 ml) was dropped on the TRG film and was then dried in the oven at 40 °C overnight. The TRG-OMo/N film was transferred into the SEM chamber and exposed to an electron beam at 2.0 kV in vacuum for 5 min to generate pores on graphene film. Instrumental characterization XRD patterns of the samples were measured from 3 to 90° by a Philips X’Pert PRO XRD instrument with CuKα ( λ =1.5418 Å) radiation (40 kV, 30 mA). SEM observations were carried out using a Hitachi S-4800 microscope (Hitachi Ltd, Japan) at an accelerating voltage of 0.5–6.0 kV. The SEM sample on carbon tape was subject to the observation without any sputter-coating. TEM observations were carried out using a Tecnai G 2 20S-TWIN microscope (FEI, USA) at an accelerating voltage of 200 kV. Samples were dispersed in ethanol and the dispersions were dropped on a copper grid and dried at 60 °C overnight. IR spectra were recorded in potassium bromide pellets using a Spectrum One Fourier transform infrared spectrometer (PerkinElmer Instruments Co. Ltd, USA). XPS data were obtained with an ESCALab220i-XL electron spectrometer (VG Scientific Ltd, UK) using 300 W AlKα radiation. The base pressure was ~3 × 10 −9 mbar. The binding energies were referenced to the C 1s line at 284.8 eV from adventitious carbon. Raman spectra were recorded with a Renishaw inVia Raman spectrometer (Renishaw plc, UK). All samples were tested in powder form on silicon wafer without using any solvent. The laser excitation was provided by a regular model laser operating at 514 nm. Nitrogen sorption isotherms were obtained with a Micromeritics TriStar II 3020 surface area and porosity analyser at 77 K. The samples were degassed overnight at 120 °C. The obtained nitrogen adsorption–desorption isotherms were evaluated to give the pore parameters, including Brunauer–Emmett–Teller specific surface area and pore volume. How to cite this article : Zhou, D. et al. A general and scalable synthesis approach to porous graphene. Nat. Commun . 5:4716 doi: 10.1038/ncomms5716 (2014).